Trends and oscillations in the Indian summer monsoon rainfall over the last two millennia Observations show that summer rainfall over large parts of South Asia has declined over the past five to six decades. It remains unclear, however, whether this trend is due to natural variability or increased anthropogenic aerosol loading over South Asia. Here we use stable oxygen isotopes in speleothems from northern India to reconstruct variations in Indian monsoon rainfall over the last two millennia. We find that within the long-term context of our record, the current drying trend is not outside the envelope of monsoon’s oscillatory variability, albeit at the lower edge of this variance. Furthermore, the magnitude of multi-decadal oscillatory variability in monsoon rainfall inferred from our proxy record is comparable to model estimates of anthropogenic-forced trends of mean monsoon rainfall in the 21st century under various emission scenarios. Our results suggest that anthropogenic-forced changes in monsoon rainfall will remain difficult to detect against a backdrop of large natural variability. Among the most serious impacts of climate change to South Asia are those that relate to water availability and drought due to changes in Indian summer monsoon (ISM) rainfall amount and spatio-temporal pattern. Although, the spatial structure of the mean seasonal rainfall over South Asia exhibits complex patterns [1] , the area-weighted all-India summer monsoon rainfall (AISMR) time series [2] serve as an adequate index of ISM intensity over continental India on interannual to decadal timescales [3] , [4] . Between AD 1870 and 1990, the AISMR appears to exhibit quasi-oscillatory multi-decadal (~60–70 years) variability, with amplitudes that are generally within ±5.0% of historical normals (~850 mm) [4] , [5] , [6] . However, in context of the last 50–60 years, the AISMR has been undergoing a statistically significant decreasing trend, which is also observed in various gridded precipitation data sets [7] , [8] , [9] . This decline stands in contrast to the near-unanimous results from climate models, which indicate increasing rainfall in a warming climate due to increasing greenhouse gas concentrations [10] , [11] . In some model simulations, the observed summertime drying trend has been attributed to increased anthropogenic aerosol loading over South Asia [8] , [9] , [12] , but considerable uncertainty remains in modelling the role of aerosols on monsoon rainfall [13] . A fundamental question therefore emerges whether the weakening of ISM rainfall, particularly over northern India (NI), is anomalous within the long-term context of natural variability. Deciphering whether the recent decade-long ISM drying trend is caused by human-induced aerosol emissions or a manifestation of ISM natural variability is critical to understanding both the near and long-term behaviour of the ISM. Although the AISMR is among the longest instrumental records of precipitation on Earth, it is still too short (~145 years) to allow a robust characterization of multi-decadal-centennial ISM variability from which, one can examine the uniqueness of the observed drying trend. Existing proxy reconstructions from South Asia suggest that the ISM exhibits complex spatio-temporal variations, the finer details of which are highlighted by speleothem oxygen isotope (δ 18 O) records from central India (CI) and northeastern India [14] , [15] , [16] , [17] , [18] . Building upon our previous work, here we present a new high-resolution and radiometric-dated speleothem δ 18 O-based reconstruction of ISM rainfall over the last two millennia. The new record is developed from two stalagmites (SAH-A and SAH-B) collected from the Sahiya Cave in NI. The climatologically unique location of our site allows us to cast temporal changes in speleothem δ 18 O in terms of decadal-averaged variations in ISM rainfall, and thus, the low-frequency aspect of our record can be construed as a paleo-counterpart of the instrumental AISMR time series. Our reconstruction reveals a wide range of ISM behaviour, consisting of multi-centennial trends forced by Northern Hemisphere (NH) temperatures, distinct multi-decadal oscillatory variability and sporadic sub-decadal intervals of anomalously high and low rainfall. Within the long-term context of our record, the observed decline in ISM rainfall since the middle of the 20th century is not outside the envelope of natural variability, albeit at the lower edge of this variance. In addition, the magnitude of ISM multi-decadal oscillatory variability inferred from our record is comparable to model estimates of anthropogenic-forced trends of mean monsoon rainfall in the 21st century under various representative concentration pathway (RCP) scenarios [11] . Our results underscore the challenge of detecting anthropogenic-forced changes in ISM against a background of large internal variability. Regional climatology The Sahiya Cave ((30°36′N, 77°52′E, ~1,190 m above sea level (m.a.s.l.)) is located ~200 km NNE of New Delhi in the Uttarakhand State of India ( Fig. 1 ; Supplementary Fig. 1 ). Mean annual temperature and annual precipitation in the region are ~22.0 °C and 1,600 mm, respectively, with ~80% of precipitation falling during the monsoon season (between June and September) ( Supplementary Fig. 2 ). The onset of ISM rainfall in the study area is preceded by the development of the cross-equatorial low-level jet (LLJ) that serves as the primary conduit for transporting moisture across the Indian Ocean and the Arabian Sea onto the Indian sub-continent [19] . The LLJ generates strong cyclonic vorticity in the planetary boundary layer (typically north of 15°N) leading to large convective instabilities over the central portion of India, a region referred to as the Monsoon Trough (MT) [20] . At the height of the ISM season (typically during July and August), the LLJ develops into a southeasterly flow, transporting moisture from the Bay of Bengal (BoB) to northwest and northern India [21] . In addition, the negative pressure anomalies in the MT region trigger the development and propagation of synoptic-scale weather systems, collectively referred to as the low-pressure systems (LPS) [20] , from the BoB (typically north of 18°N during the months of July and August) onto the Indian landmass. The LPS are instrumental in advancing the ISM as far north as the Lesser Himalayas (that is, north of our study area) and as far west as Pakistan during periods of strong monsoon circulation [21] . Another important source of precipitation variability in the study area stems from chaotic oscillations in monsoonal precipitation, referred to as active-break spells [20] , [21] , [22] . Distinct from the LPS, these oscillatory modes of monsoon exhibit a hierarchy of quasi-periods (3–7 days, 10–20 days and 30–60 days) and are manifestations of north–south fluctuations in the mean position of the MT [20] , [21] , [22] . During the ‘break’ period, the axis of the MT shifts north of our site, resulting in dry air intrusions of westerly winds into northwest and central-north India, which tend to suppress rainfall through decrease of convective instability and depletion of parcel buoyancy [23] , [24] . In summary, the sub-seasonal to interannual precipitation variability in our study area, strategically located at the distal end of the BoB branch of the ISM and at the northern periphery of the MT region, is sensitive to changes in the strength and position of the LLJ and attendant changes in the MT, which in turn, influence the strength of the BoB branch of ISM. 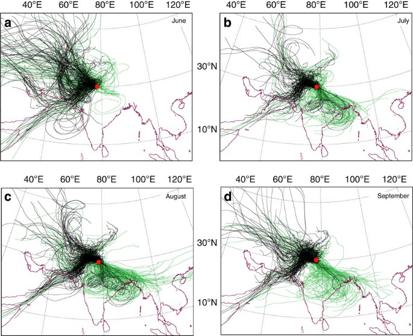Figure 1: Cave location and ensembles of backward air-parcel trajectories originating from the study area. The HYSPLIT25trajectory ensembles depict air-parcel/moisture transport routes for JJAS, highlighting the maximum contrast between strong and weak monsoon circulation. The green and black lines in each panel are multi-year monthly composites of daily trajectories originating from the study area (red dot) associated with periods of anomalously high and low rainfall, respectively, during June (a), July (b), August (c) and September (d). Anomalously low rainfall (relative to the 20th century mean) during June, July, August and September in our study area is characterized by near-cessation of18O-depleted moisture flux from the Bay of Bengal, resulting in relatively higher flux of18O-enriched moisture from the local sources and Arabian Sea, and dry air intrusions of westerly winds that tend to suppress rainfall over central and northern India through increase of convective stability. On other hand, anomalously high rainfall, particularly during July and August, in our study area is associated with significantly enhanced transport of18O-depleted moisture from the Bay of Bengal (see Methods andSupplementary Fig. 6). Figure 1: Cave location and ensembles of backward air-parcel trajectories originating from the study area. The HYSPLIT [25] trajectory ensembles depict air-parcel/moisture transport routes for JJAS, highlighting the maximum contrast between strong and weak monsoon circulation. The green and black lines in each panel are multi-year monthly composites of daily trajectories originating from the study area (red dot) associated with periods of anomalously high and low rainfall, respectively, during June ( a ), July ( b ), August ( c ) and September ( d ). Anomalously low rainfall (relative to the 20th century mean) during June, July, August and September in our study area is characterized by near-cessation of 18 O-depleted moisture flux from the Bay of Bengal, resulting in relatively higher flux of 18 O-enriched moisture from the local sources and Arabian Sea, and dry air intrusions of westerly winds that tend to suppress rainfall over central and northern India through increase of convective stability. On other hand, anomalously high rainfall, particularly during July and August, in our study area is associated with significantly enhanced transport of 18 O-depleted moisture from the Bay of Bengal (see Methods and Supplementary Fig. 6 ). Full size image Oxygen isotope in modern precipitation We use the observational data from the Global Network of Isotopes in Precipitation program of the International Atomic Energy Agency (GNIP-IAEA, hereafter GNIP) to characterize the δ 18 O of precipitation (δ 18 O p ) in our study area. The GNIP data nearest to the cave site (Uttarkashi, 30.72N, 78.44E; 1,140 m.a.s.l. ), however, contains only 3 years of monthly δ 18 O p observations (AD 2004–2006; n =28) ( Supplementary Fig. 3 ). Consequently, we use the δ 18 O p data from the GNIP station at New Delhi (28.58N, 77.52E; 212 m.a.s.l., and ~200 km south of Sahiya) to characterize the δ 18 O p variability in our study area ( Supplementary Figs 4–5 ). Our approach to utilize δ 18 O p data from New Delhi is justified by the gross similarities between the annual cycles of precipitation and δ 18 O p at Sahiya and New Delhi (see Methods), which suggest that both sites are influenced by similar precipitation dynamics and moisture sources throughout the year. Furthermore, to examine dynamical linkages between δ 18 O p and changes in the low-level (~850 hPa) monsoon circulation pattern, we use the hybrid single-particle lagrangian integrated trajectory model (HYSPLIT) [25] to generate backward (168 h) moisture trajectory ensembles for those periods where GNIP data are available. Our paired analyses of GNIP δ 18 O p data and the low-level monsoon moisture trajectory patterns ( Fig. 1 ; Supplementary Fig. 6 ) suggest that the δ 18 O p variability in the study area is dominated by large-scale changes in low-level monsoon circulation and moisture transport history upstream of our site, and to a lesser extent from changes in local precipitation intensity. We find that periods of strong (weak) monsoon circulation are characterized by an enhanced (reduced) flux of isotopically depleted BoB moisture and reduced (enhanced) flux of isotopically enriched Arabian Sea moisture to our site (see Methods). Speleothem oxygen isotope interpretation The contrasting patterns of strong and weak monsoon circulation produce distinct δ 18 O p , signatures, which in theory, should predominantly drive changes in δ 18 O of speleothems from the study area. This inference rests in part on the assumption that non-monsoon rainfall and snowmelt are insignificant sources of surface waters that infiltrate into the cave system. Indeed, this assumption is supported by the δ 18 O values of the cave’s dripwaters (−6.95±0.31‰, n =7), which are indistinguishable from the amount-weighted δ 18 O of annual precipitation (−6.97‰) and slightly higher than the δ 18 O of June, July, August and September (JJAS)-integrated precipitation (−8.19‰) in the study region ( Supplementary Fig. 3d ). Furthermore, the regional precipitation–evaporation budget is positive only during the summer monsoon season (from June to September) ( Supplementary Fig. 2b ), implying that effective infiltration of surface waters into the local karst occurs primarily during the ISM season ( Supplementary Fig. 3 ). The karstic overburden over the Sahiya Cave (~30 m) would, however, tend to act as a lowpass filter by mixing δ 18 O p signals from several seasons, thus damping high-frequency δ 18 O p variations. Nonetheless, the low-frequency (multi-year to decadal) component of the speleothem δ 18 O record should reflect time-integrated shifts in δ 18 O of karstic waters stemming from an asymmetric occurrence of 18 O-enriched (depleted) precipitation events during weak (strong) monsoon seasons. Consequently, we interpret temporal changes in the speleothem δ 18 O at our site to reflect space–time-integrated upstream changes in ISM intensity. Indeed, comparisons of the speleothem δ 18 O time series with instrumental records of precipitation at local, sub-regional and sub-continental spatial scales ( Supplementary Fig. 7 ) indicate that the strength of the inverse δ 18 O p –rainfall amount relationship is higher at sub-regional and sub-continental scales. This observation suggests that upstream changes in ISM circulation and rainfall variability rather than changes in the local precipitation amount are the primary drivers of δ 18 O variability at our site. Our observations are consistent with the results from other studies, which suggest that local δ 18 O p variability in some monsoonal and tropical regions reflect upstream changes in regional circulation and rainfall [26] , [27] . Speleothem oxygen isotope record The NI δ 18 O record from the Sahiya Cave is a composite of two δ 18 O stalagmite records (SAH-A and SAH-B) consisting of 1848 δ 18 O measurements with an average temporal resolution of 1.5 years per sample ( Supplementary Fig. 8 ). The chronologic frameworks of SAH-A and SAH-B δ 18 O profiles are provided by 13 and 15 230 Th dates, respectively ( Supplementary Fig. 9 ; Supplementary Data 1 ). The average 2 σ age uncertainty of the composite record is ~22.5 years. The age models are developed by generating multiple cubic interpolations [28] between the discrete 230 Th dates. The SAH δ 18 O record (mean=−9.0‰; 1 σ =0.24) covers the last two thousand years (BC 141 to AD 2006) ( Supplementary Data 2 ). The δ 18 O profile is characterized by prominent decadal to multi-decadal variability with an amplitude of ~0.5‰ around the long-term mean ( Fig. 2b ). The observed weakening trend in ISM rainfall since the 1950s manifests as an ~0.5‰ increase in speleothem δ 18 O, which is a robust feature of our record even with generous assumptions of age model and analytical uncertainties. Comparison between the composite δ 18 O profile and a 11-year running mean of AISMR exhibits a significant inverse correlation ( r =−0.75 with 95% confidence interval (−0.82; −0.64)) that explains ~50% of variance in the instrument record ( Fig. 2a ; Supplementary Fig. 7 ). After correcting for standard instrumental error in δ 18 O measurements (0.06‰), the slope of the speleothem δ 18 O-AISMR regression yields a conversion of 1.0‰ in speleothem δ 18 O values to ~86 mm change in AISMR, the latter equivalent to ~10% of the long-term mean (~850 mm) ( Fig. 2a ). The δ 18 O record is characterized by several episodic intervals of anomalously (>2 σ ) positive and negative δ 18 O values. Particularly noteworthy are two sub-decadal length intervals of strong pluvial and drier conditions, centred at AD ~1,100 and 1,620, respectively ( Fig. 2b ). The timing and duration of the latter event, which constitutes the largest positive δ 18 O anomalies in our reconstruction coincides (within age uncertainties) with widespread droughts and famines in north India [29] and with the collapse of the Guge Kingdom in western Tibet [30] . Incidentally, these two intervals of substantially enhanced and reduced ISM rainfall occur within the periods of peak thermal anomalies during the Medieval Climate Anomaly (nominally, AD 1000–1200) and the Little Ice Age (nominally AD ~1600–1850) ( Fig. 2 ), respectively. 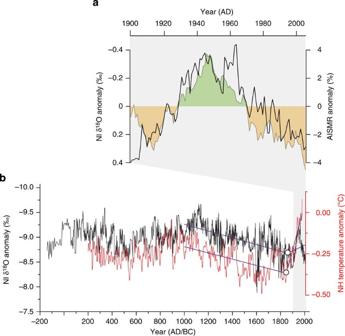Figure 2:Comparison of the NI speleothem δ18O record with instrumental and proxy data. (a) The comparison between the NI speleothem time series (raw data) shown as δ18O anomalies (relative to the mean of the time series) (black) with theyaxis reversed and the AISMR anomalies (11-year running mean) (shaded) expressed as % departure from the 20th century mean (~850 mm). (b) The NI speleothem time series shown as raw δ18O anomalies (black) and NH temperature anomalies reconstruction36(red). Bold lines (purple) are estimated trends43in the time series over the last 1,000 years. White circles mark the break points (timing of trends change). Figure 2: Comparison of the NI speleothem δ 18 O record with instrumental and proxy data. ( a ) The comparison between the NI speleothem time series (raw data) shown as δ 18 O anomalies (relative to the mean of the time series) (black) with the y axis reversed and the AISMR anomalies (11-year running mean) (shaded) expressed as % departure from the 20th century mean (~850 mm). ( b ) The NI speleothem time series shown as raw δ 18 O anomalies (black) and NH temperature anomalies reconstruction [36] (red). Bold lines (purple) are estimated trends [43] in the time series over the last 1,000 years. White circles mark the break points (timing of trends change). Full size image Spectral analysis [31] of the record reveals significant power in the 60–80- and 15–30-year bands ( Fig. 3c ). The time-frequency [32] and wavelet analyses [33] of the speleothem δ 18 O record (see Methods and Supplementary Fig. 10 ) suggest that the amplitudes of aforementioned scale-averaged oscillations are non-stationary. For example, the 60–80-year oscillatory band is dominant during the AD 300–500, 1500–1700 and 1850–2000 intervals and nearly absent during other times. Significant concentration of variance in the 60–80-year band is also common in numerous instrumental and proxy global and regional sea surface temperature (SST) records [34] . The non-stationary aspect of the ISM multi-decadal oscillatory mode likely arises from the influence of specific (and time–space varying) arrays of different modes of SST variability, which themselves are coupled in complex manners [35] . On multi-centennial and longer timescales, the δ 18 O profile over the last 1,000 years is characterized by a pronounced trend towards higher values. 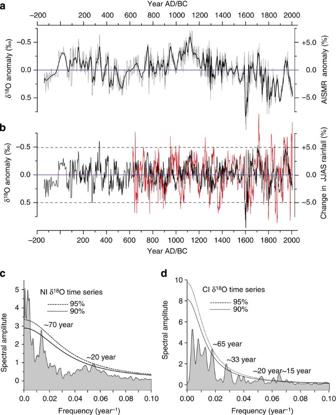Figure 3:Time series analysis of the NI and CI δ18O records. (a) The NI speleothem record shown as δ18O anomalies (relative to the mean of the time series). The δ18O anomalies are shown both as raw data (grey) and smoothed (11-year running mean) (black) along with the regressed AISMR anomalies (%). (b) The comparison between the SSA44detrended NI (black) and CI14,15,16(red) speleothem records shown as δ18O anomalies (raw data). The long-term non-stationary trends in both time series are removed by subtracting the first reconstructed component indicated by SSA of the raw data. The two dashed horizontal lines delineate a 10% change in monsoon rainfall amounts, highlighting the magnitude of multi-decadal variability inferred from our NI δ18O record. (c) Power spectrum of the composite NI and (d) CI SSA-detrended δ18O time series obtained using REDFIT31software. A varying number of Welch overlaps were used to optimize bias/variance properties. Spectral band significant above the 90% level are labelled with their period. Figure 3: Time series analysis of the NI and CI δ 18 O records. ( a ) The NI speleothem record shown as δ 18 O anomalies (relative to the mean of the time series). The δ 18 O anomalies are shown both as raw data (grey) and smoothed (11-year running mean) (black) along with the regressed AISMR anomalies (%). ( b ) The comparison between the SSA [44] detrended NI (black) and CI [14] , [15] , [16] (red) speleothem records shown as δ 18 O anomalies (raw data). The long-term non-stationary trends in both time series are removed by subtracting the first reconstructed component indicated by SSA of the raw data. The two dashed horizontal lines delineate a 10% change in monsoon rainfall amounts, highlighting the magnitude of multi-decadal variability inferred from our NI δ 18 O record. ( c ) Power spectrum of the composite NI and ( d ) CI SSA-detrended δ 18 O time series obtained using REDFIT [31] software. A varying number of Welch overlaps were used to optimize bias/variance properties. Spectral band significant above the 90% level are labelled with their period. Full size image Comparison with a central India speleothem record The Sahiya Cave δ 18 O record from NI shares key similarities and notable differences with the speleothem δ 18 O record from CI [14] , [15] , [16] (19°N and 82°E) ( Fig. 3b ; Supplementary Fig. 11 ). The latter has been shown to reflect the ISM rainfall variability over the core monsoon zone of India (defined here as ~18°–27°N and 69°–88°E). Importantly, both records exhibit strong multi-decadal variability and share common spectral power ( Fig. 3 ). Although the CI δ 18 O record has slightly larger amplitude and is more variable than the NI δ 18 O record, such differences may result, at least partially, from a varying degree of smoothing of isotopic signals imparted by processes unique to local karst at each location. The visual comparison between the two records shows similar long-term patterns but no consistent peak-to-peak relationship on decadal-multi-decadal timescales. For example, the interval with most prominent positive anomalies in the CI record (AD ~1370–1400) has no clear counterpart in the NI record, whereas the interval with most positive δ 18 O anomalies in the NI record (AD ~1600–1630) is clearly evident in the CI record ( Supplementary Fig. 11 ). While such inconsistencies may result from spatial contrast in ISM rainfall, the combined age uncertainties of both records preclude definitive assessment of phase relationships between these records on short timescales. The low-frequency (multi-centennial) aspect of our ISM reconstruction from NI is broadly similar to NH temperature reconstructions [36] over the last two millennia ( Fig. 2b ). The close correspondence between these reconstructions on such a timescale supports the notion that NH temperature is an important driver of ISM variability via changes in meridional surface/tropospheric thermal gradients [12] , [37] and the interhemispheric thermal contrast [6] , [37] . However, neither proxy nor instrumental data comparisons between ISM rainfall and NH temperatures reveal consistent relationships on decadal to multi-decadal timescales. This suggests that the thermodynamic effect on ISM rainfall maybe more important on longer timescales via changes in boundary conditions at a larger spatial scale (global or hemispherical) [37] . At shorter timescales, the ISM is more strongly influenced by changes in local and/or remote SST fields and other aspects of external boundary conditions [4] , [5] , [6] . Nonetheless, given that the magnitude of the NH temperature rise since the 1950s is unprecedented in the context of the last 2,000 years, the decreasing trend in the ISM rainfall seems anomalous in light of changes expected from a simple thermodynamical-scaling argument [38] . The latter postulates that atmospheric water vapour should increase in line with the Clausius Clapeyron relationship at ~7%°C −1 rise in atmospheric temperature due to increasing concentrations of greenhouse gases. The lack of an upward trend in ISM rainfall since the 1950s supports results from coupled climate models that include aerosol forcing [8] , [9] , [12] . These model experiments indicate that the increased anthropogenic aerosol loading over south Asia may have substantially counterbalanced a precipitation increase over continental India that would otherwise have occurred in response to singular increase in global temperatures. Parsing the relative contribution of aerosol forcing to the observed decline in ISM rainfall requires establishing an envelope of ISM baseline natural variability on decadal to multi-decadal timescales. We use the observed inverse speleothem δ 18 O–AISMR relationship in deriving, admittedly rough, quantitative estimates of decadal-scale variations in ISM. Using the standard linear regression fitted by means of the ordinary least-square method, we use the slope of the speleothem δ 18 O–AISMR relationship (~1.0‰/86 mm) to estimate decadal-scale ISM rainfall variability over the last 2,000 years ( Fig. 3 ). Although more sophisticated transfer functions employing a forward modelling approach may ultimately be more robust, any model for which the δ 18 O of monsoon precipitation (and consequently, the δ 18 O of speleothem) is inversely linked to area-weighted changes in ISM rainfall, should lead us, at least qualitatively, to the conclusion we reach as follows. Our analysis shows that the magnitude of ISM rainfall decrease since the mid-20th century is not unique in the long-term context of our record, but nonetheless right near the edge of the envelope of ISM long-term variability ( Fig. 3a ). This observation implies that the observed drying can be due to ISM natural variability alone. However, it will be imprudent to ignore the possible influence of aerosol forcing on ISM rainfall, especially considering that previous excursions to comparably drier intervals inferred from our record typically occurred in the context of cooler NH temperatures and in absence of significant human-induced aerosols emissions. It is also instructive to compare the maximum expression (peak-to-trough) of ISM multi-decadal variability in our record (~10%), for example, from AD 1720 to ~1800 ( Fig. 3b ) with anthropogenic-forced trends of mean monsoon rainfall projected from climate models for the 21st century. For example, a recent evaluation of ISM rainfall for the period 1850–2100 from 20 climate models within the Coupled Model Intercomparison Project 5 showed [11] a consistent increase in mean monsoon rainfall for the period AD 2070–2100 (relative to the historic period AD 1870–1900) under different RCP scenarios, with the highest increase in the strongest warming scenario RCP 8.5. However, only half of these models can realistically simulate the ISM [11] . The projected increase in mean ISM rainfall for the period AD 2070–2100 (relative to AD 1870–1900) from all but one of the realistic models is within 10% for all warming scenarios, which is similar to the maximum magnitude of ISM natural multi-decadal variability inferred from our record. These observations highlight the fundamental problem of detecting forced trends in ISM rainfall against the background of relatively large internal variability. Understanding the current and future changes in ISM rainfall spatio-temporal pattern and amount has enormous societal implications for more than 1.5 billion people in the region. The paleoclimate data presented here provide a baseline of ISM natural variability on multi-decadal to centennial timescales. It is on precisely these timescales that the anthropogenic-forced changes are likely to be superimposed on monsoon’s natural climate variability. Detection and attribution of climate change on ISM rainfall will require a coordinated effort through improvements in both climate models and proxy reconstructions of ISM rainfall. The paper presented here highlights the promise of this approach and provides impetus for further refinement of ISM rainfall reconstructions. Cave characteristics and sample collection In April 2007, we collected a pair of columnar-shaped stalagmites (SAH-A and SAH-B) from a small and poorly ventilated chamber, ~100 m from the cave’s entrance. The stalagmite SAH-A was found wet (and presumably actively growing) at the time of collection. In situ measurements indicate relative humidity in excess of 95%, numerous active feeder drips and a narrow range of ambient temperatures ( T cave air =21.8±0.6 °C, n =7) throughout the cave, with the latter being similar to the regional mean annual air temperature (~22.0 °C) ( Supplementary Fig. 2 ). Unlike higher altitude regions to its north, the study area (elevation ~1,000–1,200 m) does not experience snowfall. Consequently, spring snowmelt is not a source of meteoric water into the local karst above the Sahiya Cave. The regional precipitation–evaporation is positive only during the summer monsoon season ( Supplementary Fig. 2b ), suggesting that effective infiltration of meteoric waters into the local karst is only significant during the ISM season. Sample preparation The stalagmites were cut with a thin diamond blade along the growth axes. A digitally controlled triaxial micromill was used to obtain sub-samples for δ 18 O and δ 13 C analyses by continuously milling in 100-μm increments along the stalagmites growth axes, yielding sub-samples weighing typically between 100 and 130 μg for isotopic analyses. Sub-samples for 230 Th dating (weighing typically between 150 and 300 mg) were obtained by drilling with a 0.9-mm carbide dental burr. Stable isotope analysis Sub-samples for δ 18 O and δ 13 Canalyses were measured using a Multi-Prep Dual Inlet System attached to an Iso-prime Stable Isotope Ratio Mass Spectrometer at the University of Southern California. The long-term precision of the Ultissima standard for δ 18 O and δ 13 C measurements over the course of this study was ~0.06‰ and 0.03‰, respectively. Isotopic equilibrium Two lines of evidence support that calcite deposition in the Sahiya cave occurs at or near isotopic equilibrium. First, strong replication between the SAH-A and SAH-B δ 18 O records during the period of overlap ( r =0.60 with 95% confidence interval (0.17, 0.84)) ( Supplementary Fig. 8 ) suggest that both stalagmites have recorded a primary climate signal that has not been significantly altered by disequilibrium processes associated with conditions unique to each stalagmite, such as different flow pathways through the overlying bedrock, groundwater mixing and residence time, pCO 2 and so on. Second, the theoretical range of the caves’ ambient temperature (20.8–23.9 °C) under isotopic equilibrium conditions [39] calculated from the measured range in δ 18 O of dripwaters (−6.95±0.31‰, n =7) and the δ 18 O of modern calcite (−8.53‰) is well within the measured range of ambient temperature in the Sahiya cave (21.8±0.6 °C, n =7). 230 Th dating and the age model 230 Th dating was performed at the Minnesota Isotope Laboratory on a Multi-Collector Inductively Coupled Plasma Mass Spectrometer (Thermo-Finnigan Neptune). We use standard chemical procedures to separate uranium and thorium for 230 Th dating, as reported in Edwards et al . [40] The standardization and half-lives are reported in Cheng et al . [41] All U and Th isotopes were measured on a MasCom multiplier behind the retarding potential quadrupole in the peak-jumping mode. We followed similar procedures of characterizing the multiplier as described in Shen et al . [42] Initial 230 Th values were corrected and all ages are reported with a 2 σ error and are in correct stratigraphic order ( Supplementary Data 1 ). The chronologic frameworks of stalagmite SAH-A and SAH-B δ 18 O profiles are constrained by 13 and 15 230 Th dates, respectively. We use Monte Carlo simulations ( N =2,000) to account for the dating uncertainties (2.5% and 97.5% quantile confidence limits) within the time series [28] ( Supplementary Fig. 9 ; Supplementary Data 1 ). Time series analyses Confidence intervals of correlation coefficients were determined using the pairwise moving-block bootstrap method to preserve the serial dependence of time series and interval calibration to increase the accuracy [43] . To identify periodic components in the spectrum of unevenly spaced SAH-A, SAH-B and composite SAH δ 18 O time series, we applied the Lomb–Scargle Fourier transform in combination with Welch’s Overlapped Sequence Averaging procedure using the REDFIT software [31] . REDFIT produces first-order autoregressive (AR1) time series with sampling times and characteristic timescales matching those of the input climate data. A varying number of overlapping (50%) detrended segments were used to optimize bias/variance properties of spectrum estimates. The univariate spectra were bias-corrected using 1,000 Monte Carlo simulations. To assess the statistical significance of a spectral peak, REDFIT estimates the upper confidence interval of the AR1 noise for various significance levels based on a χ 2 -distribution. Temporal changes in the average amplitude of signal components were estimated using a modified harmonic-filtering algorithm [32] , which fits sinusoidal waves to an unevenly spaced series by means of least squares (analogous to the Lomb–Scargle Fourier transform). We used a sliding window of length four times the signal period and ascribe to the window’s midpoint the average signal amplitude; the window is then shifted in steps of 0.1 year. This leads to a truncation of the time interval for the resulting estimate of the average amplitude of 4 × 80/2 years=160 years, from both the lower and upper time interval bound. In addition, we also applied the conventional continuous transform wavelet analysis to annually interpolated δ 18 O data being mindful of the caveat that here interpolation might introduce artefacts, potentially biasing the derived spectra. The singular spectrum analysis-Multitaper Method (SSA-MTM) Toolkit [44] was used to remove non-stationary linear trends from the δ 18 O time series by examining the variability of the largest eigenvalue from an autocovariance matrix. SSA decomposes time series into several modes of variability (monotonic and oscillatory) and the remaining low-amplitude noise. Time series trends and associated break points (timing of trends change) are quantified using a parametric, nonlinear regression technique [43] . This model is a continuous function consisting of two linear parts that are joined at the break point. The break model is fitted to data using a weighted least-squares method with a brute-force search for the break point. Statistical uncertainties of the trend and break point are evaluated using 2,000 block bootstrap simulations, which preserve the distribution and serial dependence of the data over the length of a block. Statistical analysis of observational δ 18 O p data We extensively utilized observational monthly δ 18 O p data from two sites—Uttarkashi and New Delhi (data sets are accessible from www.naweb.iaea.org ) to characterize the δ 18 O p variability and understand the dynamical controls of the δ 18 O p –precipitation (δ 18 O p –P) relationship in our study area. The δ 18 O p data from Uttarkashi (~50 km from the Sahiya Cave) contains only 3 years of monthly δ 18 O p observations (AD 2004–2006; n =28) [45] , whereas the GNIP station at New Delhi (~200 km south of the Sahiya Cave), contains 341 monthly δ 18 O p observations (available with gaps from AD 1961 to 2008). Despite the large difference in number of observations, the annual cycles of the δ 18 O p and rainfall amount from both sites are remarkably similar ( Supplementary Fig. 2a–b ). This close correspondence is not surprising considering that both sites are under the influence of similar precipitation dynamics due to their proximity. In addition, we find strong correlation between the observational δ 18 O p data from New Delhi and simulated δ 18 O p data (extracted from the grid point nearest to the Sahiya Cave) from Experimental Climate Prediction Center’s Global Spectral Model (ECPC-GSM) fitted with isotope tracers (IsoGSM) [46] ( Supplementary Fig. 3 ). In light of these observations, we argue that the GNIP δ 18 O p database from New Delhi data can be reliably used to understand the nature of the δ 18 O p –P relationship in our study area. The New Delhi GNIP database is characterized by a large range in both monthly δ 18 O p and precipitation amount ( Supplementary Fig. 4 ). The distribution of JJAS-averaged δ 18 O p and precipitation amount illustrates a negative δ 18 O p –P relationship ( r =−0.37, with 95% confidence interval (−0.62; −0.04), n =35). The inverse δ 18 O p –P relationship for the individual months JJAS ( Supplementary Fig. 5 ) is most pronounced at the onset (June) and end (September) of the ISM season. In contrast, the inverse δ 18 O p –P relationship during the height of the monsoon season (JA) is relatively weaker despite July and August being typically the wettest months. One plausible explanation for this observation is that lower humidity, higher evaporation and unsaturated soil conditions in June and September lead to faster re-evaporation of precipitation below cloud base and from the ground, thus explaining the observed inverse δ 18 O p –P relationship through the classic amount effect. However, a critical examination of the GNIP data set, together with composite trajectory analyses of low-level monsoon winds during strong and weak monsoon seasons, suggest that sub-seasonal changes in monsoon circulation and associated changes in the moisture source and rainout history of air parcels, are more dominant contributors to the observed inverse δ 18 O p –P relationship in our study area. This can be explained as follows. The monthly observations of δ 18 O p and precipitation amount in the GNIP data exhibit a large range with some values representing extreme ends of both, δ 18 O p and rainfall amount ranges. We define the extreme values as those that fall in the lower and the upper quartiles of observed range of δ 18 O p and precipitation amount ( Supplementary Fig. 5 ). On the basis of this scheme, we classify these extreme δ 18 O p –P pairs (and their relative abundance in the GNIP database) into four groups: (a) negative-wet (NW, relatively common); (b) negative-dry (rare); (c) positive-wet (rare) and (d) positive-dry (PD, relatively common). We find that the presence or absence of the inverse δ 18 O p –P relationship is strongly sensitive to the abundance of the NW and PD pairs in the data set, and if these data pairs are removed from the regression analysis, the inverse δ 18 O p –P relationship during June weakens and vanishes for the remaining summer monsoon season. These observations suggest that the primary source of the inverse δ 18 O p –P relationship in the GNIP database arises from occurrence of anomalously strong ( 18 O depleted) and weak ( 18 O enriched) precipitation events. HYSPLIT trajectory analysis We utilized the HYSPLIT [25] model provided by the National Oceanographic and Atmospheric Administration Air Resources Laboratory together with the National Center for Environmental Prediction and National Center for Atmospheric Research Reanalysis version 1 data [47] to generate quasi-isentropic backward (168 h) trajectory ensembles of strong and weak monsoon seasons ( Fig. 1 ; Supplementary Fig. 6 ). We are cognizant that HYSPLIT-derived trajectories can have large computational errors that are inherited from uncertainties in the reanalysis products. Therefore, we increase our confidence in trajectory analysis by computing hundreds of trajectories over an extended period to identify major moisture source areas and broad circulation features that produce precipitation in our study area. For each month of the monsoon season (JJAS), we produce the ‘wet’ and ‘dry’ trajectory ensembles ( Supplementary Fig. 6 ). The ‘wet’ and ‘dry’ months are defined here as those that fall in the upper and lower quartile of the observed range in precipitation amount in the GNIP database. For each wet and dry composite, we computed ~600 isentropic back-trajectories (168 h)(sampled four times daily at UTC 00, 06, 12 and 18) initialized at 1,500 metres (above ground level corresponding to ~850 hPa). Results from a smaller sub-set of randomly selected trajectories initialized at 1.0 or 1.5 km above ground level (corresponding to ~900 and 850 hPa levels, respectively) and computed for either 120 or 168 h duration, were nearly identical. How to cite this article: Sinha, A. et al . Trends and oscillations in the Indian summer monsoon rainfall over the last two millennia. Nat. Commun. 6:6309 doi: 10.1038/ncomms7309 (2015).